Silicon-chip mid-infrared frequency comb generation Optical frequency combs are a revolutionary light source for high-precision spectroscopy because of their narrow linewidths and precise frequency spacing. Generation of such combs in the mid-infrared spectral region (2–20 μm) is important for molecular gas detection owing to the presence of a large number of absorption lines in this wavelength regime. Microresonator-based frequency comb sources can provide a compact and robust platform for comb generation that can operate with relatively low optical powers. However, material and dispersion engineering limitations have prevented the realization of an on-chip integrated mid-infrared microresonator comb source. Here we demonstrate a complementary metal–oxide–semiconductor compatible platform for on-chip comb generation using silicon microresonators, and realize a broadband frequency comb spanning from 2.1 to 3.5 μm. This platform is compact and robust and offers the potential to be versatile for use outside the laboratory environment for applications such as real-time monitoring of atmospheric gas conditions. Optical frequency combs are coherent light sources consisting of discrete lines that are equally spaced in frequency. Mid-infrared comb sources in particular have proved promising for spectroscopy as their broad bandwidth and narrow frequency linewidths make them ideal for probing narrow molecular transitions [1] . Recently, mid-infrared frequency combs have been demonstrated in a number of platforms; however, the realization of a robust on-chip integrated mid-infrared comb source has proven elusive. On-chip integration and miniaturization of the mid-infrared comb are critical, as they will enable high portability for stand-off atmospheric sensing out in the field, and as well as monolithic integration with other necessary components, such as resonant cavities for gas sensing and photodetectors for measurements. In particular, a complementary metal–oxide–semiconductor (CMOS) compatible integrated mid-infrared comb source would be inexpensive and straightforward for mass production. Mid-infrared combs have been previously demonstrated in platforms such as fibre lasers, mode-locked lasers and optical parametric oscillators [2] , [3] , [4] , but these platforms are relatively bulky and cannot be integrated. Supercontinuum generation represents another means for generating a broad spectrum in the mid-infrared and has been realized in a number of platforms including silicon waveguides [5] . However, supercontinuum generation requires a high-peak power-pulsed femtosecond source that can generate a broadband coherent spectrum, and for many applications it is desirable to have comb spacings much larger than the ~100-MHz spacing typically produced by such lasers, so that the individual comb lines can be resolved. Another route to mid-infrared comb generation is through the use of quantum cascade lasers [6] , but the active materials used make on-chip integration difficult. On-chip microresonator-based combs are promising because they can generate a broadband frequency comb in a compact and robust integrated platform but the reach of microresonator combs into the mid-infrared has been limited. With a properly phase-matched geometry, a frequency comb can be generated with a high-quality factor microresonator using a single continuous wave (CW) pump laser [7] . Using the parametric χ (3) nonlinear process of four-wave mixing, energy is transferred from the pump laser into frequency sidebands. Comb lines will be generated at modes supported by the microresonator and lead to an optical frequency comb with a spacing equal to that of the free spectral spacing of the resonant cavity. In particular, this enables microresonator combs to be engineered with line spacings in the 20–400 GHz range. Microresonator-based frequency comb sources have been demonstrated in a number of platforms, including silica, quartz, fluoride glasses, silicon nitride, Hydex glass, aluminium nitride and diamond [7] , [8] , [9] , [10] , [11] , [12] , [13] , [14] , [15] . Mid-infrared microresonator comb generation has been achieved in MgF 2 crystalline resonators, generating lines up to 2.55 μm (ref. 14 ). In particular, on-chip mid-infrared comb generation has not been realized because of the difficulty of creating a highly confined and high-quality factor microresonator in semiconductor thin films. Even though silicon, owing to its CMOS compatibility, wide transparency window and high third optical nonlinearity, is an ideal platform for on-chip comb generation deep into the mid-infrared, its linear and nonlinear losses have until now prevented the realization of a silicon microresonator-based comb source. Silicon has a wide-transparency window from 1.2 μm to past 8 μm (ref. 16 ) and a large third-order optical nonlinearity ( n 2 =10 −14 cm 2 W −1 at 2.5 μm wavelength [17] ), which makes it an excellent platform for mid-infrared nonlinear optics. In etched silicon microresonators, quality factors have been limited by scattering losses because of roughness in the waveguide sidewalls, which is made worse by the high index contrast between waveguide core and cladding. The dominant nonlinear loss in silicon in the 2.2–3.3 μm region is three photon absorption (3PA)—a process where three photons are simultaneously absorbed to excite an electron-hole pair [18] . The number of photons lost directly to 3PA is small (dominated by linear waveguide losses), but the generated free-carrier population will induce significant optical losses [19] . Here we overcome both silicon’s high-linear and nonlinear losses to demonstrate a proof-of-principle silicon microresonator frequency comb source, and to show the fabrication techniques necessary to achieve an on-chip integrated microresonator comb source in the mid-infrared. Design and fabrication of silicon resonators We overcome silicon’s linear losses using a novel etchless fabrication process based on thermal oxidation to achieve a high-quality factor of 590,000 in a silicon microresonator at a wavelength of 2.6 μm. The silicon waveguide is defined in an etchless manner using thermal oxidation, instead of dry etching, to form the waveguide core [20] , [21] . We deposit low-pressure chemical vapour deposition silicon nitride on top of a 500-nm silicon-on-insulator wafer. The silicon nitride serves as an oxidation mask. We then pattern and etch only the silicon nitride, and then thermally oxidize the wafer. The silicon underneath the nitride mask does not oxidize, leaving the silicon waveguide core intact. This method avoids the roughness and absorption sites that can be introduced by reactive ion etching [22] . This method is particularly useful here, due to the need for a silicon slab for electrical integration. As the slab surface is never etched, we avoid the high losses typically associated with active silicon resonators. We characterize the resonator quality factor by sweeping a narrow linewidth source across the resonance, and measuring the transmission spectrum using a 10-MHz photodiode. The transmission spectrum is shown in Fig. 1b . The loaded quality factor is 220,000 and the intrinsic one is 590,000, which corresponds to a propagation loss of 0.7 dB cm −1 . See Methods for full fabrication process. 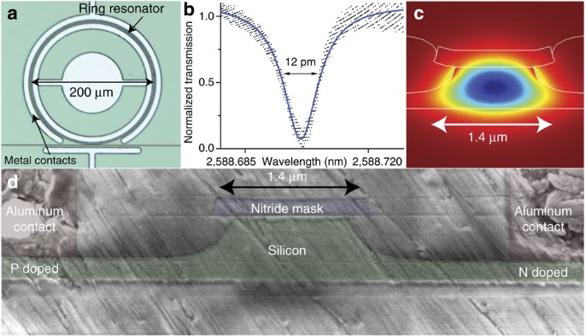Figure 1: Profile of the etchless silicon microresonator with integrated PIN diode. (a) Optical microscope image of a ring resonator and metal contacts fabricated using the etchless process. (b) Normalized transmission spectrum taken at low-input power, showing an overcoupled resonance with an intrinsic quality factor of 590,000. (c) Simulated optical mode at 2.6 μm, showing high-modal confinement in Si. (d) False coloured cross-sectional SEM image of silicon waveguide, doped regions and metal contacts. Figure 1: Profile of the etchless silicon microresonator with integrated PIN diode. ( a ) Optical microscope image of a ring resonator and metal contacts fabricated using the etchless process. ( b ) Normalized transmission spectrum taken at low-input power, showing an overcoupled resonance with an intrinsic quality factor of 590,000. ( c ) Simulated optical mode at 2.6 μm, showing high-modal confinement in Si. ( d ) False coloured cross-sectional SEM image of silicon waveguide, doped regions and metal contacts. Full size image To enable broadband comb generation, we engineer the etchless waveguide geometry to have anomalous group velocity dispersion from 2.2 to 3 μm. The geometry of the silicon waveguide governs the bandwidth of the frequency comb as the waveguide cross-section determines its dispersion profile [9] , [23] . The simulated group velocity dispersion is shown in Fig. 2a . We use the commercial software Silvaco Athena to simulate the oxidation process, to obtain the waveguide profile. From repeated tests, we have found good agreement between the simulated waveguide profile and the actual etchless waveguide formed. The simulated bandwidth for a frequency comb generated in this geometry is shown in Fig. 2b , for 150 mW of optical power in the bus waveguide and an assumed 10 ps free-carrier lifetime. To simulate the spectral-temporal dynamics of the microresonator combs, we use a recently developed numerical approach [23] , [24] based on the Lugiato-Lefever equation [25] , [26] . Here we modify the method to take into account multi-photon absorption and the free-carrier dynamics on the generated optical spectra. This adds additional loss terms (free-carrier and 3PA) to the Lugiato-Lefever equation, as well as a term for the dispersive effects of the free-carriers. With the free-carrier population kept at low levels (10 ps lifetime), simulations predict that generation of a coherent frequency comb in this geometry is possible (see Supplementary Note 1 ). 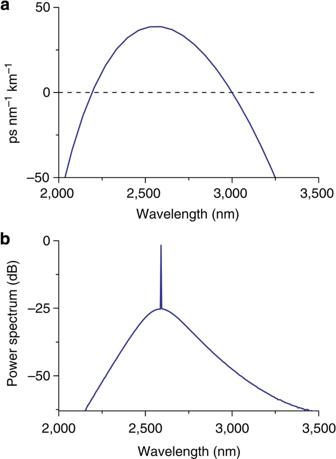Figure 2: Dispersion engineering and simulated comb bandwidth for the silicon microresonator. (a) Group velocity dispersion for the etchless silicon waveguide. We achieve broad anomalous dispersion from 2.2 to 3.0 μm in a silicon waveguide with 1,400nm × 500 nm cross-sectional dimensions. (b) Simulated comb bandwidth with 150 mW of optical pump power in the bus waveguide, assuming a 10-ps free-carrier lifetime. Figure 2: Dispersion engineering and simulated comb bandwidth for the silicon microresonator. ( a ) Group velocity dispersion for the etchless silicon waveguide. We achieve broad anomalous dispersion from 2.2 to 3.0 μm in a silicon waveguide with 1,400nm × 500 nm cross-sectional dimensions. ( b ) Simulated comb bandwidth with 150 mW of optical pump power in the bus waveguide, assuming a 10-ps free-carrier lifetime. Full size image To mitigate silicon’s nonlinear loss, we embed the silicon microresonator in a reverse biased positive-intrinsic-negative (PIN) doped junction to sweep out carriers generated from three-photon absorption. Significant free-carriers accumulate when pumping a passive silicon waveguide with a CW laser, limited only by the natural free-carrier lifetime of the structure. Here, we counteract the carrier generation while using a CW pump by extracting the generated carriers using a PIN junction operated in reverse bias [27] . The PIN junction prevents the electrical injection of carriers into the waveguide while allowing generated free carriers to be swept out—with effective free-carrier lifetimes demonstrated as short as 12 ps (ref. 28 ). Generation of silicon mid-infrared frequency comb We demonstrate the generation of an optical frequency comb between 2.1 and 3.5 μm under reverse bias conditions. We use as our source an Argos Model 2400 CW optical parametric oscillator, which is tunable from 2,500 to 3,200 nm with a 100-kHz linewidth. We couple 1.2 W of optical power at 2.59 μm into a lens, which focuses the light into a silicon nanotaper on the chip. The input coupling loss is roughly 9 dB, leading to 150 mW of optical power coupled into the bus waveguide on the chip. By tuning into resonance from the short wavelength side, we achieve a soft thermal lock [29] , where cavity heating is compensated by diffusive cooling to maintain constant power in the resonator. Once on resonance, we extract 2.7 mA of current, using 10 V of reverse bias applied to the PIN junction. This relatively high current is an indication that three-photon absorption is significant at these power levels. We collect the output light from the nanotaper using another lens, and couple this light to a Fourier transform infrared spectrometer (FTIR). We use a Thorlabs OSA205 FTIR for our measurements. The generated frequency comb has a uniform line spacing of 127±2 GHz, well below the 7.5-GHz resolution limit of the FTIR. This corresponds well with the expected free spectral range of the resonator. We measure an oscillation threshold with a low power of 3.1±0.6 mW in the bus waveguide, consistent with a simulation predicted threshold on the order of 10 mW. To resolve the full extent of the frequency comb and overcome the limited dynamic range for the FTIR, we filter the output lines using a series of optical bandpass filters. These filters attenuate the pump and the central part of the comb, allowing us to reach the noise floor of the FTIR. The comb spectrum as shown in Fig. 3 is then corrected for the spectral profile of the filters. 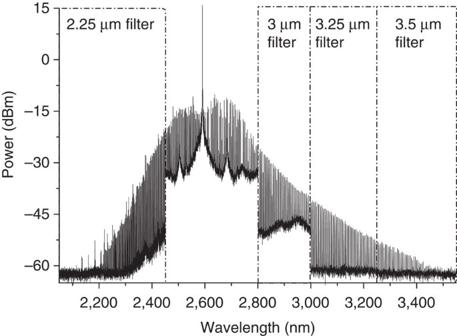Figure 3: Mid-infrared optical frequency comb generation from an etchless silicon microresonator. Broadband frequency comb generation from 2.1 to 3.5 μm in the etchless silicon micro-resonator. This frequency comb is generated with 150 mW of optical power in the bus waveguide, and with a 10-V reverse bias applied on the PIN junction. The frequency spacing of the comb is 127 GHz. Owing to the limited dynamic range of the optical spectrum analyser, the frequency comb was measured using a series of optical filters. Figure 3: Mid-infrared optical frequency comb generation from an etchless silicon microresonator. Broadband frequency comb generation from 2.1 to 3.5 μm in the etchless silicon micro-resonator. This frequency comb is generated with 150 mW of optical power in the bus waveguide, and with a 10-V reverse bias applied on the PIN junction. The frequency spacing of the comb is 127 GHz. Owing to the limited dynamic range of the optical spectrum analyser, the frequency comb was measured using a series of optical filters. Full size image We observe a strong influence on the comb spectral shape from the voltage applied to the diode, indicating that control of the carrier population through the PIN diode is critical for broadband comb generation. Without carrier extraction, frequency comb generation is limited by the natural free-carrier lifetime of the waveguide—which we measured to be 5.23±0.83 ns. See Methods for details. To test the effect of carrier extraction, we tune into resonance and fix the wavelength of our pump. At this detuning with the PIN completely off, only a few comb lines are generated above the experimental noise floor, as shown in Fig. 4a . The broad peaks at 2,510 and 2,685 nm are artefacts of the FTIR. By increasing the voltage, we find that we can dramatically increase the number of comb lines being generated: the number of comb lines above the noise floor increases from a few to hundreds, as seen in Fig. 4b . Here we can see that the initial comb lines have cascaded, showing the formation of minicombs every 50 nm. At higher voltages, these will fill in completely (see Fig. 3 ). 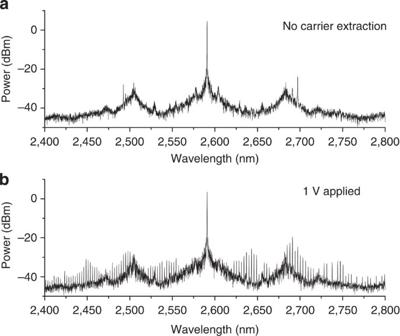Figure 4: Investigation of the effect of carrier extraction on frequency comb generation. The effect of three photon absorption on frequency comb generation depends strongly on the bias voltage of the PIN structure. The broad peaks at 2,510 and 2,685 nm are artefacts of the FTIR. (a) With the pump set at a fixed wavelength and the voltage source off, only a few lines are generated near 2,500 and 2,700 nm at this detuning. (b) By applying even a small voltage in reverse bias to the junction, we can generate hundreds of comb lines across the spectrum. Figure 4: Investigation of the effect of carrier extraction on frequency comb generation. The effect of three photon absorption on frequency comb generation depends strongly on the bias voltage of the PIN structure. The broad peaks at 2,510 and 2,685 nm are artefacts of the FTIR. ( a ) With the pump set at a fixed wavelength and the voltage source off, only a few lines are generated near 2,500 and 2,700 nm at this detuning. ( b ) By applying even a small voltage in reverse bias to the junction, we can generate hundreds of comb lines across the spectrum. Full size image In summary, we have demonstrated an on-chip integrated mid-infrared frequency comb source using an etchless silicon microresonator and demonstrated parametric oscillation in a silicon platform. We have shown electrical control of the frequency comb profile by varying the carrier extraction voltage. The etchless silicon microresonator comb source operates with low pump power well within the typical output of semiconductor laser diodes making it compatible with on-chip integration of the pump laser. An important next step is to experimentally investigate the noise and coherence properties of the generated spectra [30] , [31] , as well as the effect of free-carrier population on those properties. This platform enables a versatile and straightforward source for mid-infrared gas spectroscopy and opens the door for compact and robust mid-infrared gas sensors. The ability to achieve comb generation in an integrated platform will enable practical realization of completely integrated mid-infrared comb-based spectrometers usable in a myriad of environments. Device fabrication A thermal oxidation-based ‘etchless’ fabrication process was used to fabricate the devices. Using a commercial silicon-on-insulator wafer with a 500-nm silicon layer and a 3-μm buried oxide, 200 nm of silicon nitride was deposited using low-pressure chemical vapour deposition. Electron beam lithography was used to pattern the nitride layer, using ma-N-2405 electron-beam resist. The silicon nitride mask was patterned 1.4 μm for the waveguide layer. The ring resonator is 100 μm bending radius, with a 1.2-μm-long straight section at the coupling region. The gap between the waveguide and ring is 500 nm. After exposure and development, the silicon nitride was etched in fluorine chemistry. The wafer was then thermally oxidized at 1,200 °C to form the etchless waveguide structure. The wafer was oxidized for 20, 50 and 60 min of dry, wet and dry oxidation, respectively. The slab in the taper region was then etched away. The taper was patterned to be 350 nm wide. The wafer was then clad with 2 μm of plasma-enhanced chemical vapour deposition silicon dioxide. The oxide was then etched away next to the waveguides, and then the slab was doped with boron and phosphorous on either side to form a PIN diode. Finally, the wafer was metalized, and wires were patterned and etched. Free-carrier lifetime measurement For carrier lifetime measurements, we perform pump-probe experiments with a counter-propagating pulsed pump and CW probe. An Erbium-doped fibre laser (1,550 nm, 500 fs full-width half-maximum) is amplified to a peak power of ~200 W in an erbium-doped fibre amplifier, then coupled via a circulator into one facet of the chip. A CW probe (1,575 nm) is coupled into the opposite facet and appears on the third port of the circulator, isolated from the pump. Neither laser overlaps with a ring resonance; we measure only the bus waveguide. We further improve probe isolation by wavelength filtering the third port output with a grating filter, then route this fibre to an optical sampling oscilloscope. The oscilloscope is triggered off the pump laser’s fast sampling photodiode, giving us a time-domain measurement of the transmission of the waveguide after strong pump excitation. Absorption increases sharply when the pump-generated free-carriers flood the waveguide, then exponentially decreases as they recombine. We take the time constant of this exponential to be the free-carrier lifetime. How to cite this article: Griffith, A. G. et al . Silicon-chip mid-infrared frequency comb generation. Nat. Commun. 6:6299 doi: 10.1038/ncomms7299 (2015).